A genetic variant of p53 restricts the mucous secretory phenotype by regulating SPDEF and Bcl-2 expression Despite implications for carcinogenesis and other chronic diseases, basic mechanisms of p53 and its variants in suppressing Bcl-2 levels are poorly understood. Bcl-2 sustains mucous cell metaplasia, whereas p53 −/− mice display chronically increased mucous cells. Here we show that p53 decreases bcl-2 mRNA half-life by interacting with the 5′ untranslated region (UTR). The p53– bcl-2 mRNA interaction is modified by the substitution of proline by arginine within the p53 proline-rich domain (PRD). Accordingly, more mucous cells are present in primary human airway cultures with p53 Arg compared with p53 Pro . Also, the p53 Arg compared with p53 Pro displays higher affinity to and activates the promoter region of SAM-pointed domain-containing Ets-like factor (SPDEF), a driver of mucous differentiation. On two genetic backgrounds, mice with targeted replacement of prolines in p53 PRD show enhanced expression of SPDEF and Bcl-2 and mucous cell metaplasia. Together, these studies define the PRD of p53 as a determinant for chronic mucous hypersecretion. The importance of Bcl-2 and its family members in cell survival, differentiation and oncogenesis has been demonstrated extensively. Bcl-2 overexpression inhibits cell death and can promote cell transformation when present together with mutations of certain oncogenes [1] , [2] . For example, combined expression of Bcl-2 and c-Myc leads to the rapid transformation of lymphocytes and other cell types [3] , [4] . Consistent with its oncogenic function, Bcl-2 is aberrantly overexpressed in a wide range of human tumours, including B-cell and T-cell lymphomas [5] and non-small cell lung carcinomas [6] . This central gate-keeping role of Bcl-2 necessitates a highly controlled regulation of its expression. Despite its functional importance, the molecular mechanisms regulating Bcl-2 expression are largely unknown. We and others have reported on evidence that p53 affects transcriptional activity of a partial Bcl-2 promoter in pulmonary epithelial cells [7] , [8] , [9] , which was consistent with numerous studies reporting that p53 acts as a transcription factor [10] . The bcl-2 gene is composed of three exons whereby exons 1 and 2 are separated by a long intron of 150 kb (ref. 11 ). Exon-1 contains the 5′ up-stream region with promoters P1 and P2 and part of the protein coding open reading frame (ORF) [12] . Exon-2 encodes for parts of the ORF and the 3′UTR, and the remainder of which is encoded by exon 3. The P2 promoter region contains a CCAAT box and a TATA element and is the primary suppressor of the P1 promoter. This negative regulatory region is highly conserved across species and may be modulated by the M region of the bcl-2 promoter [7] . Our previous studies show that pulmonary inflammation initiates airway epithelial cell proliferation and Bcl-2 expression in proliferating epithelial cells [13] , [14] . Gain- and loss-of-function studies showed that Bcl-2 expression sustains hyperplastic epithelial cells, and Bcl-2 expression is elevated in airway mucous cells of subjects with cystic fibrosis [15] , in patients with chronic mucous hypersecretion (CMH) [16] and in airway epithelium of asthmatics [17] . Chronic obstructive pulmonary disease (COPD) encompasses a spectrum of diseases, with chronic bronchitis (CB) at one end and emphysema at the other. The classic definition for CB is chronic cough and sputum production for at least 3 months per year for two consecutive years [18] , although it is not clear whether CB is a disease of large airways only or whether inflammation in small airways causes mucous cell metaplasia that plays a distinct role in the development of CB. Although all smokers develop an inflammatory response, CB is only observed in a subset of heavy smokers [19] , and in approximately half of these individuals CB persists even after quitting smoking [20] . Smokers with CB are at higher risk of increased exacerbation rate [21] , longer recovery period following acute COPD exacerbations [22] , worse health-related quality of life including general health status, severe respiratory symptoms, increased physical activity limitation [23] and have worse lung function [24] . In addition, among subjects with COPD, those with CB are at higher risk for accelerated decline in lung function [25] and lung cancer [26] , [27] , and are prone to increased mortality [22] , especially after lung volume reduction surgery [28] . Persistent CB in former smokers may be due to some intrinsic factors such as susceptibility genes that predispose them to this condition. Therefore, intervention strategies for reducing CB requires identification of endogenous factors including genetic polymorphisms that make smokers susceptible to sustained CMH. In the present study, we show that when Bcl-2 regulation is analysed in the context of the entire promoter construct, p53 primarily regulates Bcl-2 levels by reducing the mRNA half-life rather than affecting promoter activity. When studying the detailed mechanisms of p53-induced suppression of Bcl-2 regulation and how that may affect the role of sustaining metaplastic mucous cells, we determined that two p53 variants, due to a polymorphism at codon 72, differentially affect bcl-2 mRNA half-life and are associated with increased CB in smokers. In addition, microarray expression analysis of primary human airway epithelial cells (HAECs) homozygote for the two genotypes pointed to the differential regulation of SPDEF, a protein that is sufficient and necessary to drive the mucous regulatory phenotype in airway cells. Both the high mucous secretory phenotype and increased Bcl-2 and SPDEF levels were also observed in mice when the highly conserved proline-rich domain of p53, where the corresponding human variant resides, was modified. Together, these studies provide the fundamental understanding of CMH and may help not only the detection and early management of this debilitating disease but also the development of effective therapies. Absence of p53 prolongs mucous cell metaplasia Our previous studies have shown that Bcl-2 is expressed in metaplastic mucous cells in various animal models of CB and asthma [13] , [14] , [29] . Furthermore, we have shown that Bcl-2 sustains metaplastic mucous cells [15] and that p53 is involved in regulating Bcl-2 expression [7] . To investigate whether the regulation of Bcl-2 by p53 translates into modification of mucous cell metaplasia, the extent of mucous cell metaplasia (MCM) in airway epithelia at airway generations 3, 4 and 5 was quantified in p53 +/+ and p53 −/− mice at 5, 8 and 12 days, respectively, after intranasal instillations of lipopolysaccharide (LPS). In p53 +/+ mice the numbers of mucous cells per mm basal lamina were increased at 5 and 8 days post instillation and returned to baseline at 12 days ( Fig. 1a ). However, in p53 −/− mice MCM remained elevated at 12 days and was higher than that observed in p53 +/+ at the same time point ( Fig. 1a ). Immunostaining of lung tissue sections from p53 +/+ and p53 −/− mice at 12 days post LPS instillation showed that Bcl-2 and Muc5ac positivity was significantly higher in p53 −/− mice ( Fig. 1b ) both when quantified as percentage of total epithelial cells or as numbers per mm basal lamina ( Fig. 1c,d ). These results suggest that Bcl-2 expression was sustained in p53 −/− mice causing persistent MCM, while Bcl-2 was downregulated in p53 +/+ mice allowing the resolution of MCM at 12 days. 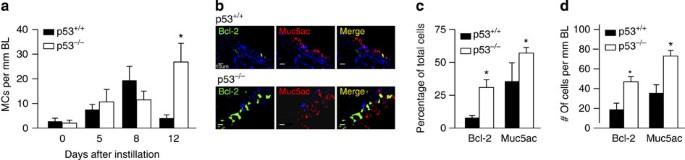Figure 1: MCM is sustained longer inp53−/−compared withp53+/+mice. (a)p53+/+andp53−/−were instilled with LPS and MCM was quantified after 5, 8 and 12 days of instillation. MC per mm basal lamina is reduced inp53+/+but is sustained inp53−/−mice at 12 days following LPS instillation. (b) Lung tissue sections fromp53+/+andp53−/−mice at 12 days post instillation were immunostained with antibodies to Bcl-2 and Muc5ac and with DAPI to visualize nuclei (scale bar 10 μm). (c) Percentages for Bcl-2- and Muc5ac-positive cells. (d) Cell numbers of Bcl-2- and Muc5ac-positive cells per millimeter basal lamina. Bar=group means±s.e.m. (n=3–5 mice/group); *P<0.05. Figure 1: MCM is sustained longer in p53 −/− compared with p53 +/+ mice. ( a ) p53 +/+ and p53 −/− were instilled with LPS and MCM was quantified after 5, 8 and 12 days of instillation. MC per mm basal lamina is reduced in p53 +/+ but is sustained in p53 −/− mice at 12 days following LPS instillation. ( b ) Lung tissue sections from p53 +/+ and p53 −/− mice at 12 days post instillation were immunostained with antibodies to Bcl-2 and Muc5ac and with DAPI to visualize nuclei (scale bar 10 μm). ( c ) Percentages for Bcl-2- and Muc5ac-positive cells. ( d ) Cell numbers of Bcl-2- and Muc5ac-positive cells per millimeter basal lamina. Bar=group means±s.e.m. ( n =3–5 mice/group); * P <0.05. Full size image p53 affects bcl-2 mRNA levels and stability Several studies have documented a suppressive effect of p53 on Bcl-2 (refs 8 , 9 ) and an inverse correlation of p53 and Bcl-2 levels for squamous lung cancers [30] . Consistent with these reports, the p53-sufficient H23 and AALEB cells showed reduced bcl-2 mRNA and protein levels compared with p53-deficient SAOS-2 cells ( Supplementary Fig. 1A, B ). These results were further confirmed in p53-deficient SAOS-2 cells stably expressing p53 or the respective controls ( Supplementary Fig. 1C ) and in H1299 cells that were stably transfected with a temperature-sensitive form of p53 (H1299p53 ts ) ( Supplementary Fig. 1D ). Similarly, HCT116 cells deficient in p53 ( Fig. 2a ) and primary murine airway epithelial cells (MAECs) from p53 −/− mice ( Fig. 2d ) expressed increased bcl-2 mRNA levels compared with the respective wild-type controls. 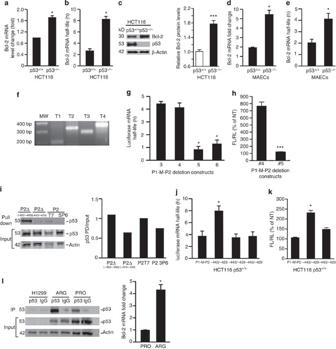Figure 2: p53 reduces Bcl-2 protein and mRNA levels by destabilizingbcl-2mRNA. (a)Bcl-2mRNA levels inp53+/+andp53−/−HCT116 quantified by qRT-PCR. (b)Bcl-2mRNA half-life inp53+/+andp53−/−HCT116 cells determined after DRB treatment for 0, 2, 4, 6 and 8 h and Bcl-2 mRNA quantified by qRT-PCR. (c) Bcl-2 protein levels inp53+/+andp53−/−HCT116 cells with densitometric quantification normalized to actin content shown in the lower panel. (d)Bcl-2mRNA levels and mRNA half-life (e) inp53−/−andp53+/+primary mouse airway epithelial cells (MAECs). (f) RT-PCR for T1, T2, T3 and T4bcl-2transcripts of HAECs. (g) Luciferase mRNA half-life analysed in H1299p53tscells transfected with P1MP2-Δ3, Δ4, Δ5 and Δ6 -luciferase constructs, treated with DRB at 16 h post transfection and RNA collected at 0, 2, 4 and 6 h. (h) Luciferase activity for P1MP2-Δ4 and Δ5 constructs measured using firefly (FL) to renilla (RL) luciferase ratio. (i) The P2 region cloned in the pCRII dual promoter vector was used to generate Bio-11-UTP-labelled sense and anti-sense RNA using the T7 and Sp6 promoters, respectively; the labelled RNAs were pull-down using H1299p53tsS-100 cytosolic extracts. p53 was detected in pull-down products using sense (lane 3) but not anti-sense RNA (lane 4). Bio-11-UTP-labelled sense RNA prepared from two deletions introduced into the P2-containing constructs—pCR-II P2(−482/−468) and pCR-II P2(−443/−429). Pull-down assays performed with sense RNA from pCR-II P2(−482/−468) (lane 1), pCR-II P2(−443/−429) (lane 2). Densitometric quantification of pull-down products normalized to the input shown in left panel. (j) Luciferase mRNA half-life for P1MP2Δ(−443/−429, −443/−439, −433/−429) luciferase and wild-type P1MP2 luciferase vectors following transfection into HCT116 p53+/+cells (k) The luciferase activity for wild-type P1MP2 luciferase and P1MP2Δ−443/−439, −433/−429) luciferase constructs. (l) Cell extracts prepared from H1299 and H1299p53ts cells maintained at 32 °C were immunoprecipitated using anti-p53 or IgG1and probed for p53 on a western blot. Analysis of pull-down products forbcl-2mRNA by qRT-PCR was normalized to the total protein and input. Bars=group means±s.e.m. (n=3 different treatments/group); *P<0.05; ***P<0.0001. Figure 2: p53 reduces Bcl-2 protein and mRNA levels by destabilizing bcl-2 mRNA. ( a ) Bcl-2 mRNA levels in p53 +/+ and p53 −/− HCT116 quantified by qRT-PCR. ( b ) Bcl-2 mRNA half-life in p53 +/+ and p53 −/− HCT116 cells determined after DRB treatment for 0, 2, 4, 6 and 8 h and Bcl-2 mRNA quantified by qRT-PCR. ( c ) Bcl-2 protein levels in p53 +/+ and p53 −/− HCT116 cells with densitometric quantification normalized to actin content shown in the lower panel. ( d ) Bcl-2 mRNA levels and mRNA half-life ( e ) in p53 −/− and p53 +/+ primary mouse airway epithelial cells (MAECs). ( f ) RT-PCR for T1, T2, T3 and T4 bcl-2 transcripts of HAECs. ( g ) Luciferase mRNA half-life analysed in H1299p53 ts cells transfected with P1MP2-Δ3, Δ4, Δ5 and Δ6 -luciferase constructs, treated with DRB at 16 h post transfection and RNA collected at 0, 2, 4 and 6 h. ( h ) Luciferase activity for P1MP2-Δ4 and Δ5 constructs measured using firefly (FL) to renilla (RL) luciferase ratio. ( i ) The P2 region cloned in the pCRII dual promoter vector was used to generate Bio-11-UTP-labelled sense and anti-sense RNA using the T7 and Sp6 promoters, respectively; the labelled RNAs were pull-down using H1299p53 ts S-100 cytosolic extracts. p53 was detected in pull-down products using sense (lane 3) but not anti-sense RNA (lane 4). Bio-11-UTP-labelled sense RNA prepared from two deletions introduced into the P2-containing constructs—pCR-II P2(−482/−468) and pCR-II P2(−443/−429). Pull-down assays performed with sense RNA from pCR-II P2(−482/−468) (lane 1), pCR-II P2(−443/−429) (lane 2). Densitometric quantification of pull-down products normalized to the input shown in left panel. ( j ) Luciferase mRNA half-life for P1MP2Δ(−443/−429, −443/−439, −433/−429) luciferase and wild-type P1MP2 luciferase vectors following transfection into HCT116 p53 +/+ cells ( k ) The luciferase activity for wild-type P1MP2 luciferase and P1MP2Δ−443/−439, −433/−429) luciferase constructs. ( l ) Cell extracts prepared from H1299 and H1299p53ts cells maintained at 32 °C were immunoprecipitated using anti-p53 or IgG 1 and probed for p53 on a western blot. Analysis of pull-down products for bcl-2 mRNA by qRT-PCR was normalized to the total protein and input. Bars=group means±s.e.m. ( n =3 different treatments/group); * P <0.05; *** P <0.0001. Full size image We previously observed that the P2 promoter region of the bcl-2 gene, when analysed alone or in the absence of P1 or M regions, interacts with and was suppressed by p53 (ref. 7 ). To further evaluate the effect of p53 on P2 promoter activity in the context of the full-length promoter that contains the P1, M and P2 regions, we compared the promoter activities of constructs containing the progressively deleted P2 region in p53-sufficient A549 and p53-deficient H1299 cells ( Supplementary Table 1 ). The activities of the P1-M-P2 promoter were lower in both cells lines when >140 bp of the P2 region was present ( Supplementary Fig. 2A ). Similarly, when the same constructs were tested in H1299 cells stably transfected with the temperature-sensitive p53 (p53 ts ), the P2 region effectively reduced promoter activity regardless of the p53 activation status ( Supplementary Fig. 2B ). The promoter activity assays repeatedly showed that p53 minimally suppressed bcl-2 promoter activity, and removal of the entire P2 region affected promoter activity only by a factor of 2–3. In fact, promoter activity appeared to be increased when p53 was activated at 32 °C ( Supplementary Fig. 2B ). These findings did not adequately explain the >10-fold suppression of Bcl-2 expression by p53. To further evaluate the reason for reduced Bcl-2 levels in p53-sufficient cells, we investigated whether p53 may affect bcl-2 mRNA stability. Bcl-2 mRNA half-life was significantly longer in the p53-deficient H1299 and SAOS-2 cells compared with the p53-sufficent A549 and AALEB cells ( Supplementary Fig 2C ). The effect of p53 was further confirmed by the observation that bcl-2 mRNA half-life was longer in p53 −/− HCT116 cells and in primary MAECs from p53 −/− mice compared with the p53 +/+ counterparts ( Fig. 2b,e and Supplementary Fig. 2D,E ). This shorter half-life in bcl-2 mRNA translated into lower Bcl-2 protein levels in p53-sufficient and p53-deficient HCT116 cells ( Fig. 2c ). Together, these results showed that p53 enhances the degradation of bcl-2 mRNA. p53 interacts with the P2 region within the 5′UTR of bcl-2 mRNA Although the role of p53 as a transcriptional regulator is extensively studied, the role of p53 in regulating mRNA stability is unknown. As p53 affected bcl-2 mRNA stability and p53 interacted with the P2 region, we investigated whether this region is part of the 5′UTR of bcl-2 mRNA. As mechanisms involving immortalization can introduce possible artefacts in cell lines, we investigated whether the 5′UTR also extends to the P1 region by preparing bcl-2 RNA from primary HAECs and mapping the transcriptional start sites using 5′RACE. Primers designed to amplify various regions within the 5′UTR identified four different transcriptional start sites: T1, T2, T3 and T4. Sequence analysis revealed that T1 and T2 originate within the P1 region at −1,778 and −1,313, respectively ( Supplementary Fig. 3A ). T3 and T4 were localized within the P2 region of bcl-2 gene, and transcriptional start sites were mapped to nucleotides −465 and −176 upstream of the ORF, respectively ( Supplementary Fig. 3A ). To further validate the findings from the 5′RACE, we used primers specific to either P2 or M regions for RT-PCR using DNase-treated RNA that was isolated from various epithelial cell lines. Both sets of primers successfully amplified products specific to the P2 ( Supplementary Fig. 3B ) and M ( Supplementary Fig. 3C ) regions in RNA isolated from AALEB and SAOS-2 cell lines. These findings further confirmed that P2 sequences are part of the Bcl-2 transcript not only in primary cells, but also in other cell types assayed, including cancer cells. We also investigated whether P2 sequences are transcribed when they are present as promoter-luciferase constructs in which sequences representing the 3′UTR are excluded. The P2 and M regions were detected by RT-PCR in A549 and H1299 cells that were transfected with luciferase constructs containing P1-M-P2 or P2 promoter regions using forward primers specific for P2 or M and luciferase cDNA-specific reverse primers ( Supplementary Fig. 3D–F ). Collectively, our findings confirmed that sequences of P2 region are represented within the 5′UTR of Bcl-2 transcripts in several cell lines and that the absence of 3′UTR sequences of bcl-2 mRNA did not affect the transcriptional start site of bcl-2 gene. In addition, the bcl-2 transcripts for T1, T2, T3 and T4 were successfully amplified by RT-PCR using specific primers designed within the 5′UTR ( Fig. 2f ). These results demonstrate that p53 interacts with the bcl-2 transcripts and suggest that P2 sequences on bcl-2 mRNA could represent sites of interaction with p53. As our results demonstrated that P2 sequences are part of bcl-2 mRNA 5′UTR, we next investigated whether p53 interacts with bcl-2 mRNA. A P2 region mediates p53-dependent destabilization of bcl-2 mRNA The interaction of p53 with the 5′UTR suggested that the P2 region is responsible for the p53-dependent degradation of bcl-2 mRNA. Previous findings have reported that the critical region for p53 interaction with the Bcl-2 promoter lies within P2 region [7] , [8] , [31] . To identify 5′UTR sequences within bcl-2 mRNA that are responsible for p53-dependent bcl-2 mRNA decay, HCT116p53 +/+ cells were transfected with P1-M-P2 luciferase constructs that contain progressive deletions within P2 ( Supplementary Information , Supplementary Table 1 ). Luciferase mRNA half-life ( Fig. 2g and Supplementary Fig. 2F ) and luciferase activity ( Fig. 2h ) were reduced drastically from ~4.5 h in P1-M-P2Δ4 to ~1–2 h in P1-M-P2Δ5 construct, suggesting that the deleted 66 nucleotides (regions −423 to −489) in P1-M-P2Δ5 were important for p53-dependant RNA degradation. To confirm that the 66-nucleotide region interacts with p53, we first conducted RNA pull-down assays using in vitro transcribed bcl-2 mRNA. For this purpose, we subcloned the P2 fragment into the PCR2.1 dual promoter vector to generate sense and anti-sense biotinylated mRNAs and found that p53 was only detected in pull-down products using sense mRNA ( Supplementary Fig. 3G ). Hence, interaction of p53 with bcl-2 mRNA was confirmed by both p53 antibody and bcl-2 mRNA pull-downs. These results were confirmed by in vitro RNA pull-down assays using a short synthetic 50-nucleotide construct that comprises nucleotides −443/−429. To further delimit the site of interaction, mutations were introduced by changing the first or second 8 nucleotides or by modifying the 16 nucleotides in sets of 4 nucleotides (representing the 16 nucleotides in P2−443/−429) to random sequences as shown in Supplementary Table 2 . All of the mutations disrupted p53 interaction with this region because in vitro RNA prepared from a control nucleotide sequence within the P2 region (−608/−582) did not show p53 binding suggesting that the interaction is specific to these 16-nucleotide sequence ( Supplementary Fig. 3H ). To further characterize the sequences within the 66-nucleotide region that interact with p53, two deletion mutants, P2Δ−482/−468 and P2Δ−443/−429, were generated using site-directed mutagenesis. RNA pull-down assays using these deletion mutants revealed that the 16 nucleotides (−443/−429) were important for the interaction with p53 ( Fig. 2i ). To determine the influence of these nucleotides on mRNA half-life in vivo , we deleted the corresponding sequence in P1-M-P2 to generate P1-M-P2Δ(−443/−429)-luciferase construct and compared the luciferase mRNA half-life following transfection of HCT116p53 +/+ cells. The luciferase mRNA half-life ( Fig. 2j and Supplementary Fig. 2G ) and luciferase activity were increased by approximately twofold ( Fig. 2l ) for the P1-M-P2 compared with the P1-M-P2Δ(−443/−429) luciferase constructs, respectively, suggesting that p53 must interact with these sequences to destabilize the mRNA. Furthermore, introducing four nucleotide mutations at loci −443/−439 and −433/−429 within the P1-M-P2-luciferase construct did not affect luciferase mRNA half-life ( Fig. 2j and Supplementary Fig. 2G ), suggesting that merely mutating four nucleotides is not sufficient to completely abrogate the interaction of p53 in cells. Overall, these results show that the 16-nucleotide region within P2 is crucial for the interaction of p53 with the bcl-2 mRNA. This reduction in bcl-2 mRNA half-life by p53 Pro suggests that the PRD of p53 plays an important role in this decay process. To further study the possible differences in the interaction of p53 Arg and p53 Pro with bcl-2 mRNA, we performed a pull-down assay using a p53 antibody or IgG 1 as control from H1299 parent cells, H1299p53 ts Arg and H1299p53 ts Pro cells. p53 was absent in the parent H1299 cells and bcl-2 mRNA was greater in pull-down products from H1299p53 ts Arg compared with H1299p53 ts Pro cells even when normalizing for the reduced p53 Pro levels detected in the pull-down products ( Fig. 2l ), supporting the idea that p53 Arg has a higher affinity to the bcl-2 mRNA than p53 Pro . Genetic variation in p53 is associated with chronic bronchitis As Bcl-2 sustains mucous cells that may be responsible for increased mucous hypersecretion in chronic diseases, such as cystic fibrosis [15] and CB [29] , we wanted to investigate whether the differential regulation of Bcl-2 by p53 could be associated with increased CMH in humans. First, we tested whether we can identify single-nucleotide polymorphisms (SNPs) within the 5′UTR of Bcl-2 mRNA that affects p53-dependant RNA degradation and Bcl-2 expression. We sequenced the highly conserved P2 region in 200 individuals from the Lovelace Smokers Cohort (LSC) and were unable to identify SNPs within this highly conserved region. As p53 has a SNP at codon 72 (rs1042522) that modifies the common amino acid, arginine encoded by CGC, to a proline encoded by CCC, we next tested the idea whether the two p53 variants affect the interaction with 5′UTR sequences within bcl-2 mRNA. The Pro at codon 72 constitutes the second of the five PXXP (where P indicates proline and X indicates any amino acid) within the proline-rich domain (aa 61–94) [32] , [33] , and two independent cohort studies had found that the p53 Pro variant is associated with attenuated decline in lung function in humans [25] , [34] . Because of the finding that p53 is a critical regulator of bcl-2 mRNA and the resolution of MCM, we tested whether polymorphisms within p53 may be associated with CMH in the LSC. Initially, we genotyped participants of the LSC when only 1,102 women were enrolled of whom 370 participants had CMH as defined by having self-reported cough and productive phlegm for 3 months a year for at least two consecutive years [35] and 732 did not. Of the 1,102 women, 77 (7%) were homozygous p53 Pro , 606 (55%) homozygous p53 Arg and 419 (38%) heterozygous p53 Arg/Pro . We found that after adjusting for age and smoking duration, subjects who are homozygous for the rare p53 Pro allele had a significantly reduced odds for CB compared with those with the p53 Arg genotype (OR=0.48, P =0.03). The p53 PRD is important for interaction with bcl-2 mRNA To investigate whether the p53 SNP affects bcl-2 mRNA half-life and to possibly identify the domain in p53 that interacts and destabilizes bcl-2 mRNA, we compared bcl-2 mRNA levels and half-lives in three HAECs individually each homozygous for the p53 Arg and p53 Pro variants. We found that after averaging the bcl-2 mRNA levels in HAECs with the p53 Arg variant (HAEC Arg ) were approximately twofold greater than that in p53 Pro HAECs ( Fig. 3a ). Bcl-2 mRNA half-life was >10 h in primary HAECs, irrespective of genotype, when p53 was not activated but following activation of p53 by irradiating these cells to 10 mJ UV light; bcl-2 mRNA half-life was reduced to 1.2 h in HAEC Pro and to 7 h in HAEC Arg cells ( Fig. 3b ). This reduction in bcl-2 mRNA half-life by p53 Pro suggests that the PRD of p53 plays an important role in this decay process. Bcl-2 protein levels were also reduced in HAEC Pro compared with HAEC Arg cells ( Fig. 3c ). 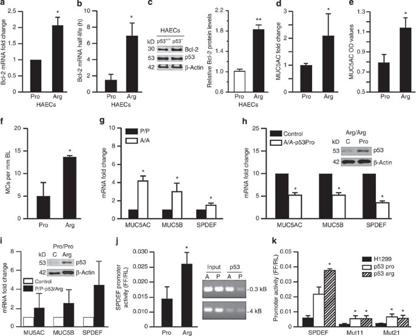Figure 3: p53Arginteracts and upregulates SPDEF to stimulate the mucous regulatory network. (a) Bcl-2 mRNA levels in primary HAECArgand HAECProcultures. (b) Bcl-2 mRNA half-life in primary HAECs 2 h after activating p53 by exposing cells to 10 mJ UV. HAECs from three individuals with p53Argor the p53Provariants were treated with DRB and Bcl-2 mRNA half-life was determined at 0, 2, 4, 6 and 8 h. (c) Bcl-2 protein levels in HAECArgand HAECProcells with densitometric quantification normalized to actin content shown in the lower panel. (d) Comparison of MUC5AC mRNA levels by qRT-PCR in HAECArgand HAECProcultures from 10 individuals each. HAECs were differentiated on ALI cultures. (e) MUC5AC protein in washes from HAECArgand HAECProcultures from 10 individuals each determined by ELISA. (f) The number of mucous cells per mm basal lamina determined by counting cells using morphometry. (g) Validation of expression of MUC5AC, MUC5B and SPDEF mRNAs by qRT-PCR based on microarray results from HAECArgand HAECProcultures from 10 individuals each. (h) Expression of p53Proin HAECArgcells using adenoviral expression vector reduces expression of MUC5AC, MUC5B and SPDEF. (i) Expression of p53Argin HAECProcells using adenoviral expression vector increases expression of MUC5AC, MUC5B and SPDEF. (j) SPDEF promoter in pGL3Basic exhibits a higher promoter activity in the H1299tsArg cells compared with H1299tsPro cells. (k) ChIP assay using p53 antibodies from H1299tsArg and H1299tsPro cells showed that significantly more DNA was pulled down from the Arg cells compared with the Pro cells. Input denotes that similar DNA amounts were used for the pull-down experiment. Interaction of p53 is visible when using primers specific to the −0.3 kB region but absent when using primers specific to the −4 kB region. (l) H1299, H1299tsArg and H1299tsPro cells transfected with promoter constructs for SPDEF, deletion mutant 11 and deletion mutant 12 in pGL3Basic and promoter activities were measured. Promoter activity was reduced for both cell types with both mutants. Bars=group means±s.e.m. (n=3 different treatments/group); *P<0.05; **P<0.001. Figure 3: p53 Arg interacts and upregulates SPDEF to stimulate the mucous regulatory network. ( a ) Bcl-2 mRNA levels in primary HAEC Arg and HAEC Pro cultures. ( b ) Bcl-2 mRNA half-life in primary HAECs 2 h after activating p53 by exposing cells to 10 mJ UV. HAECs from three individuals with p53 Arg or the p53 Pro variants were treated with DRB and Bcl-2 mRNA half-life was determined at 0, 2, 4, 6 and 8 h. ( c ) Bcl-2 protein levels in HAEC Arg and HAEC Pro cells with densitometric quantification normalized to actin content shown in the lower panel. ( d ) Comparison of MUC5AC mRNA levels by qRT-PCR in HAEC Arg and HAEC Pro cultures from 10 individuals each. HAECs were differentiated on ALI cultures. ( e ) MUC5AC protein in washes from HAEC Arg and HAEC Pro cultures from 10 individuals each determined by ELISA. ( f ) The number of mucous cells per mm basal lamina determined by counting cells using morphometry. ( g ) Validation of expression of MUC5AC, MUC5B and SPDEF mRNAs by qRT-PCR based on microarray results from HAEC Arg and HAEC Pro cultures from 10 individuals each. ( h ) Expression of p53 Pro in HAEC Arg cells using adenoviral expression vector reduces expression of MUC5AC, MUC5B and SPDEF. ( i ) Expression of p53 Arg in HAEC Pro cells using adenoviral expression vector increases expression of MUC5AC, MUC5B and SPDEF. ( j ) SPDEF promoter in pGL3Basic exhibits a higher promoter activity in the H1299 ts Arg cells compared with H1299 ts Pro cells. ( k ) ChIP assay using p53 antibodies from H1299 ts Arg and H1299 ts Pro cells showed that significantly more DNA was pulled down from the Arg cells compared with the Pro cells. Input denotes that similar DNA amounts were used for the pull-down experiment. Interaction of p53 is visible when using primers specific to the −0.3 kB region but absent when using primers specific to the −4 kB region. ( l ) H1299, H1299 ts Arg and H1299 ts Pro cells transfected with promoter constructs for SPDEF, deletion mutant 11 and deletion mutant 12 in pGL3Basic and promoter activities were measured. Promoter activity was reduced for both cell types with both mutants. Bars=group means±s.e.m. ( n =3 different treatments/group); * P <0.05; ** P <0.001. Full size image To test whether the HAEC Pro would also express less mucous compared with HAEC Arg cells, we identified 10 HAEC each from individuals homozygous for p53 Pro and p53 Arg and differentiated them individually in culture over 21 days at air–liquid interface (ALI) on Transwell membranes. When averaged, MUC5AC mRNA levels in these cultures were significantly lower in HAEC Pro compared with HAEC Arg ( Fig. 3d ). In addition, HAEC Pro cultures exhibited less secreted mucous ( Fig. 3e ) and mucous cells per mm basal lamina compared with HAEC Arg cultures ( Fig. 3f ). These results showed that the p53 Pro and p53 Arg genotypes affected the mucous phenotype. Codon 72 polymorphism affects the mucous regulatory network In airway epithelial cells, increased survival per se is not sufficient to provide the mucous differentiation phenotype, suggesting that p53 Arg may be controlling genes that affect the mucous differentiation pathway. Therefore, we isolated RNA from 10 each differentiated HAEC Pro and HAEC Arg cultures and interrogated all expressed genes by microarray analysis. One of the genes found to be expressed at significantly lower levels in HAEC Pro compared with HAEC Arg cultures was SPDEF. From the list of genes identified to be differentially expressed, we focused on SPDEF, because it has recently been described as being a transcription factor sufficient to cause goblet cell differentiation of Clara cells [36] and as a regulator of the transcriptional network mediating the goblet cell differentiation and mucous hyperproduction associated with chronic pulmonary disorders [37] . Differences in expressed genes were validated using qRT-PCR and showed that expression of MUC5AC, MUC5B and SPDEF was reduced in HAEC Pro compared with HAEC Arg cultures ( Fig. 3g ). In addition, using adenoviral expression vectors forced expression of p53 Pro in HAEC Arg cultures from three individuals significantly reduced expression of MUC5AC, MUC5B and SPDEF mRNAs ( Fig. 3h ), while expression of p53 Arg in HAEC Pro cultures from three individuals increased expression of these genes reversing the endogenous levels of these mRNAs ( Fig. 3i ). In addition, suppression of Bcl-2 or SPDEF using retroviral shRNA vectors reduced MUC5AC mRNA levels in HAEC Arg cultures ( Supplementary Fig. 4A–D ). These findings further demonstrated that it is the genotype of p53 that determined expression of genes driving the mucous regulatory phenotype. While Bcl-2 may sustain hyperplastic mucous cells, we assumed that SPDEF may be responsible for the differentiation of the HAEC Arg cultures to express the mucous phenotype. Therefore, we investigated whether the promoter region of SPDEF may be driven differently by two p53 variants to cause the observed differences in mucous differentiation of HAECs. We identified two putative p53 response elements within 1 kb upstream of the SPDEF transcriptional start site and cloned this region into pGL3 Basic containing a luciferase reporter and tested activation in H1299 ts Arg and H1299 ts Pro cells. Following transfection with the luciferase construct and activation of the temperature-sensitive p53 by shifting cells from 37° to 32 °C for 18 h, the SPDEF promoter activity was consistently twofold lower in p53 Pro versus p53 Arg cells ( Fig. 3j ). These findings suggested that p53 Arg has a higher affinity to the SPDEF promoter. Therefore, we performed chromatin immunoprecipitation (ChIP) assays using p53 antibodies and found that the 0.3 kB region of the SPDEF promoter was recovered at significantly higher levels from H1299 ts Arg compared with H1299 ts Pro cells ( Fig. 3k ). The 4 kB upstream region was used as a negative control and showed little interaction in both cell lines ( Fig. 3l ). These findings confirmed that p53-SPDEF promoter binding exhibited a significantly higher affinity in H1299 ts Arg versus H1299 ts Pro cells. The p53 response element is defined by two canonical decamers separated by a spacer of 0–13 nucleotides [38] . The SPDEF promoter region contained two (RRRCWWGYYY) motifs with a four-nucleotide spacer. As the core region (CWWG) is critically important for p53 binding [38] , deletion mutations were generated by removing six nucleotides for each of the two motifs in the core region to form two different 6 NT deletions termed Mut11 and Mut21. The empty plasmid, Mut11, and Mut21 constructs when tested in the parental H1299, H1299 ts Arg and H1299 ts Pro cell lines showed that while p53 Arg is better than p53 Pro in activating the wild-type promoter, SPDEF promoter activity was significantly reduced in both Arg and Pro cell lines when the core regions of the p53 response elements were absent ( Fig. 3k ). These findings confirmed that p53 activated SPDEF promoter by interacting with these conserved response elements. Susceptibility to death in cells harbouring p53 Arg or p53 Pro Bcl-2 suppresses DNA damage-induced cell death [39] . As p53 Pro drastically reduced bcl-2 mRNA stability, we investigated whether cell death is enhanced in p53 Pro -expressing cells that are grown in the presence of mRNA synthesis inhibitors and various cell death stimuli. When treated with the DNA damaging agent, doxorubicin (Dox), H1299p53 ts Pro cells were more sensitive to the DNA damage than H1299p53 ts Arg cells, but not to cycloheximide (CHX)- or thapsigargin (TG)-induced cell death ( Fig. 4a ). 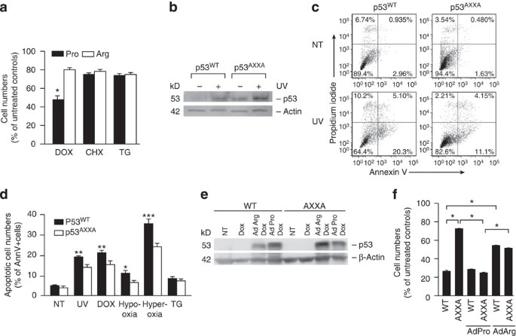Figure 4: The proline-rich domain of p53 affects DNA damage-induced cell death in airway epithelial cells. (a) H1299p53tsArg and H1299p53tsPro cells treated with 50 ng ml−1DRB, and 1 μM doxorubicin, 10 μM cyclohexamide or 1 μM thapsigargin, and cell numbers quantified 48 h later. (b) p53 levels were increased in p53WTand p53AXXAMEFs when treated with 10 mJ UV irradiation. (c) p53WTand p53AXXAMEFs treated with 10 mJ UV irradiation in the presence of 50 ng ml−1DRB and cell death analysed by Annexin V and propidium iodide (PI) staining. (d) Quantification of Annexin V-positive cells in p53WTand p53AXXAMEFs following treatment for 8 h with 50 ng ml−1DRB and either 10 mJ UV irradiation, 1 μM doxorubicin, 5% O2(hypoxia), 95% O2(hyperoxia) or 1 μM thapsigargin. (e) Western blot verifying the presence of p53 after infection of p53WTand p53AXXAMEFs with adenoviral vectors expressing p53Argor p53Pro. (f) p53WTand p53AXXAMEFs were either left untreated (control) or infected with adenoviral vectors for p53Argor p53Prothen treated with 1 μM doxorubicin for 24 h and cell numbers quantified. Bars=group means±s.e.m. (n=3 different treatments/group); *P<0.05; **P<0.01; ***P<0.0001. Figure 4: The proline-rich domain of p53 affects DNA damage-induced cell death in airway epithelial cells. ( a ) H1299p53 ts Arg and H1299p53 ts Pro cells treated with 50 ng ml −1 DRB, and 1 μM doxorubicin, 10 μM cyclohexamide or 1 μM thapsigargin, and cell numbers quantified 48 h later. ( b ) p53 levels were increased in p53 WT and p53 AXXA MEFs when treated with 10 mJ UV irradiation. ( c ) p53 WT and p53 AXXA MEFs treated with 10 mJ UV irradiation in the presence of 50 ng ml −1 DRB and cell death analysed by Annexin V and propidium iodide (PI) staining. ( d ) Quantification of Annexin V-positive cells in p53 WT and p53 AXXA MEFs following treatment for 8 h with 50 ng ml −1 DRB and either 10 mJ UV irradiation, 1 μM doxorubicin, 5% O 2 (hypoxia), 95% O 2 (hyperoxia) or 1 μM thapsigargin. ( e ) Western blot verifying the presence of p53 after infection of p53 WT and p53 AXXA MEFs with adenoviral vectors expressing p53 Arg or p53 Pro . ( f ) p53 WT and p53 AXXA MEFs were either left untreated (control) or infected with adenoviral vectors for p53 Arg or p53 Pro then treated with 1 μM doxorubicin for 24 h and cell numbers quantified. Bars=group means±s.e.m. ( n =3 different treatments/group); * P <0.05; ** P <0.01; *** P <0.0001. Full size image In mice, the PRD consists of two PXXP motifs highly resembling human p53. Mice expressing p53 lacking the four critical proline residues at loci 79, 82, 84 and 87 that make up the tandem PXXP sites (p53 AXXA ) were generated to study the role of the PRD in Mdm2-mediated degradation of p53 (refs 40 , 41 ). The p53 AXXA mice develop normally and the transcriptional activation of target genes, apoptosis induction [41] or acetylation [42] are not impaired. MEFs from p53 WT and p53 AXXA mice showed comparable rate of proliferation in culture. We first subjected cultured MEF cells to UV light and determined that the mutation of the PXXP motif to AXXA of the PRD does not prevent stabilization of p53 protein by western blotting ( Fig. 4b ). Analysis of the dying cells revealed that when treated with Dox the MEF WT compared with MEF AXXA cells showed a higher percentage of Annexin V-and PI-positive cells at 8 h ( Fig. 4c ). MEFs from p53 wt mice were more susceptible to Dox-, UV irradiation-, hypoxia- or hyperoxia-induced cell death than p53 AXXA MEFs, especially in the presence of the transcription inhibitor, DRB, at 8 h ( Fig. 4d ) and at 18 h ( Supplementary Fig. 6A,B ) after treatment with cell death inducers. However, MEFs were equally sensitive to thapsigargin (TG)- ( Fig. 4d ) or cycloheximide (CHX)-induced cell death ( Fig. 4d and Supplementary Fig. 6 ). These findings suggest that when transcription is blocked, enhanced degradation of bcl-2 mRNA by the p53 Pro variant makes cells more susceptible to DNA damage-induced cell death compared with cells in which the PRD is modified resulting in a longer half-life and higher bcl-2 mRNA levels. This was also true in the absence of the transcriptional inhibitor where in p53 AXXA MEFs cell death was significantly reduced compared with p53 wt MEFs. Further, p53 wt and p53 AXXA MEFs were infected with adenoviral vectors expressing p53 Arg and p53 Pro and then treated with Dox. Western blotting following infection with Ad-p53 Arg and Ad-p53 Pro showed that similar levels were expressed ( Fig. 4e ). However, cell death in MEFs was significantly increased when infected with Ad-p53 Pro and, as expected, p53 wt MEFs gained resistance to cell death when infected with Ad-p53 Arg ( Fig. 4f ). These findings further confirm that the p53 Pro variant enhances decay of the anti-apoptotic Bcl-2 and thereby sensitizes cells to Dox-induced cell death. PRD of murine p53 also affects the mucous regulatory network To determine whether the two PXXP motifs or the two threonines affect mRNA stability, we compared bcl-2 mRNA stability in MAECs and MEFs from wild-type p53 (p53 wt ), p53 AXXA and p53 ΔP mice. Bcl-2 mRNA levels were higher in mutant alleles versus wild type in MEFs ( Fig. 5a ) and MAECs ( Fig. 5d ), and mRNA half-life was increased from 1.5 to ~5 h in MEFs ( Fig. 5b and Supplementary Fig. 2I ) and 2 to ~4 h in MAECs ( Fig. 5e and Supplementary Fig. 2J ) from p53 wt and p53 AXXA mice, respectively, following activation of p53 with 10 mJ UV radiation. Bcl-2 protein levels were also increased in MEFs ( Fig. 5c ) and MAECs ( Fig. 5f ) from p53 AXXA compared with p53 WT mice. These results confirm that the murine p53 PRD, similar to the human p53 PRD, is crucial in affecting bcl-2 mRNA decay. Furthermore, the studies in murine cells show that modifying not only the prolines but also the threonines within the p53 PRD to alanines equally increased bcl-2 mRNA levels. 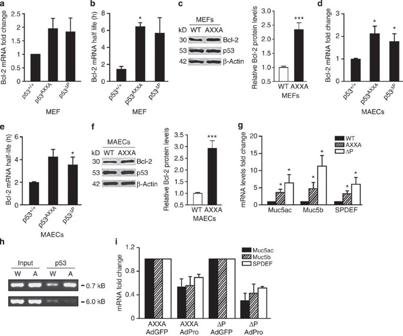Figure 5: The proline-rich domain of murine p53 regulatesbcl-2mRNA levels and half-life, and the expression of mucous differentiation genes. Bcl-2mRNA levels (a,d) and mRNA half-life (b,e) in MEFs (a,b) and in MAECs (d,e), respectively, from p53WT, p53ΔPand p53AXXAmice after treatment with 10 mJ UV light was determined after treating with DRB and collecting RNA samples at 0, 2, 4, 6, 8, 10 and 12 h for analysis by qRT-PCR. Experiments were repeated at least three times with each experiment containing 3–4 independent repeats. Bcl-2 protein levels in MEFs (c) and MAECs (f) from p53WTand p53AXXAmice with densitometric quantification of Bcl-2 protein levels normalized to actin content shown in the lower panels. (g) MAECs isolated from p53WT, p53AXXAand p53ΔP/ΔPmice were differentiated on air-liquid interface cultures on Transwell membranes and RNA analysed by qRT-PCR forMuc5ac,Muc5bandSPDEF. (h) ChIP assay using p53 antibodies from p53WTand p53AXXAMEFs showed that significantly more DNA was pulled down from the AXXA cells compared with the WT cells. Input denotes that similar DNA amounts were used for the pull-down experiment. Interaction of p53 is visible when using primers specific to the −0.7 kB region but absent when using primers specific to the −6 kB region. (i) p53AXXAand p53ΔPMAECs were differentiated on air-liquid interface cultures and infected with adenoviruses AdGFP (control) and AdPro. Isolated RNA was analysed by qRT-PCR forMuc5ac,Muc5bandSPDEF. Bars=group means±s.e.m. (n=3 different treatments/group); *P<0.05; ***P<0.0001. Figure 5: The proline-rich domain of murine p53 regulates bcl-2 mRNA levels and half-life, and the expression of mucous differentiation genes. Bcl-2 mRNA levels ( a , d ) and mRNA half-life ( b , e ) in MEFs ( a , b ) and in MAECs ( d , e ), respectively, from p53 WT , p53 ΔP and p53 AXXA mice after treatment with 10 mJ UV light was determined after treating with DRB and collecting RNA samples at 0, 2, 4, 6, 8, 10 and 12 h for analysis by qRT-PCR. Experiments were repeated at least three times with each experiment containing 3–4 independent repeats. Bcl-2 protein levels in MEFs ( c ) and MAECs ( f ) from p53 WT and p53 AXXA mice with densitometric quantification of Bcl-2 protein levels normalized to actin content shown in the lower panels. ( g ) MAECs isolated from p53 WT , p53 AXXA and p53 ΔP/ΔP mice were differentiated on air-liquid interface cultures on Transwell membranes and RNA analysed by qRT-PCR for Muc5ac , Muc5b and SPDEF . ( h ) ChIP assay using p53 antibodies from p53 WT and p53 AXXA MEFs showed that significantly more DNA was pulled down from the AXXA cells compared with the WT cells. Input denotes that similar DNA amounts were used for the pull-down experiment. Interaction of p53 is visible when using primers specific to the −0.7 kB region but absent when using primers specific to the −6 kB region. ( i ) p53 AXXA and p53 ΔP MAECs were differentiated on air-liquid interface cultures and infected with adenoviruses AdGFP (control) and AdPro. Isolated RNA was analysed by qRT-PCR for Muc5ac , Muc5b and SPDEF . Bars=group means±s.e.m. ( n =3 different treatments/group); * P <0.05; *** P <0.0001. Full size image As mucous levels increase in those individuals harbouring the p53 Arg variant, we investigated whether changes in murine PRD also affect expression of the mucous regulatory network. Mice with a deletion of the PRD (p53 ΔP ) or expressing p53 lacking the four critical proline residues at loci 79, 82, 84 and 87 that make up the tandem PXXP sites (p53 AXXA ) were generated to study the role of the PRD in Mdm2-mediated degradation of p53 (refs 40 , 41 ). MAECs isolated from wild type, p53 AXXA and p53 ΔP mice and differentiated on ALI cultures showed increased levels in SPDEF, Muc5ac and Muc5b mRNAs compared with the p53 wt MAECs ( Fig. 5g ). As MEFs express comparable levels of SPDEF transcripts as MAECs ( Supplementary Fig. 6C ), we conducted a ChIP assay to determine whether similar to the human cells p53 may interact with the murine SPDEF promoter region. A 0.7-kB region of the murine SPDEF promoter was recovered at significantly higher levels from p53 AXXA compared with p53 WT MEFs ( Fig. 5h ). A 6-kB upstream region was used as a negative control and showed no interaction in p53 AXXA and p53 WT MEFs ( Fig. 5h ). These findings confirmed that the murine SPDEF promoter also interacts with p53 and that replacing the prolines with alanines significantly increased affinity to the promoter region. Further, we infected MAECs from p53 AXXA and p53 ΔP mice with adenoviral expression vector for GFP (Ad-GFP) or p53 Pro (Ad-p53 Pro ) to test whether the p53 Pro is protective from increased mucous production. Cells were allowed to differentiate in ALI cultures and analysed for SPDEF, Muc5ac and Muc5b mRNAs levels. Levels of these mRNAs were reduced when these cells were infected with Ad-p53 Pro versus Ad-GFP ( Fig. 5i ). These findings further define the role of p53 Pro variant as being protective from increased mucous production. Another mouse strain in which threonines 76 and 86 were mutated to alanines (p53 TTAA ) was generated to remove putative Pin1 binding sites [41] . As modification of the PRD within p53 appeared to modify the regulation of SPDEF and Bcl-2 and the human epidemiological data indicated that the p53 variants was associated with CB, we investigated expression of Muc5ac and Muc5b in the lung tissues not only of p53 wt , p53 AXXA and p53 ΔP mice but also of p53 TTAA mice. Consistent with findings in human studies, increased Muc5b ( Fig. 6a ) and Muc5ac ( Fig. 6b ) mRNA levels were more pronounced in mice with mutations in the PRD compared with wild-type mice. 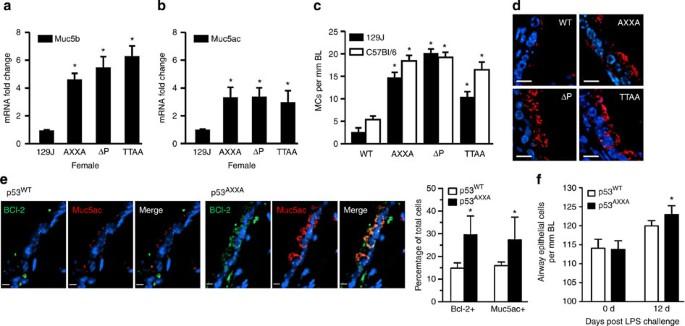Figure 6: The proline-rich domain of p53 is crucial in regulating mucous differentiation. RNA from the right cranial lung lobes of p53WT, p53AXXAand p53ΔPmice were analysed by qRT-PCR for Muc5b (a) and Muc5ac (b). (c) Mucous cells per mm basal lamina were quantified in the axial airways of p53WT, p53AXXA, p53ΔPand p53TTAAmice on 129J and C57Bl/6 backgrounds. Bars=group means±s.e.m. (n=6 mice/group); * denotes statistically significant difference. (d) Representative micrographs of airway tissue sections from p53WT, p53AXXA, p53ΔPand p53TTAAmice on 129J immunostained for Muc5ac (red) and counterstained with DAPI (blue) for nuclear staining. Scale bar, 10 μm. (e)p53WTandp53AXXAmice were instilled with LPS and changes in Bcl-2- and Muc5ac-positive cells was quantified after 12 days of instillation. Representative micrographs from p53WTand p53AXXAmice airway sections at 12 days post LPS instillation showing the Bcl-2 (green) and Muc5ac (red) immunostained cells and with DAPI (blue) nuclear counterstaining. Scale bar, 5 μm. (f) Total airway epithelial cell numbers per millimeter basal lamina at 0 days (baseline) and at 12 days post LPS instillation. Bars=group means±s.e.m. (n=>3 mice/group); *P<0.05. Figure 6: The proline-rich domain of p53 is crucial in regulating mucous differentiation. RNA from the right cranial lung lobes of p53 WT , p53 AXXA and p53 ΔP mice were analysed by qRT-PCR for Muc5b ( a ) and Muc5ac ( b ). ( c ) Mucous cells per mm basal lamina were quantified in the axial airways of p53 WT , p53 AXXA , p53 ΔP and p53 TTAA mice on 129J and C57Bl/6 backgrounds. Bars=group means±s.e.m. ( n =6 mice/group); * denotes statistically significant difference. ( d ) Representative micrographs of airway tissue sections from p53 WT , p53 AXXA , p53 ΔP and p53 TTAA mice on 129J immunostained for Muc5ac (red) and counterstained with DAPI (blue) for nuclear staining. Scale bar, 10 μm. ( e ) p53 WT and p53 AXXA mice were instilled with LPS and changes in Bcl-2- and Muc5ac-positive cells was quantified after 12 days of instillation. Representative micrographs from p53 WT and p53 AXXA mice airway sections at 12 days post LPS instillation showing the Bcl-2 (green) and Muc5ac (red) immunostained cells and with DAPI (blue) nuclear counterstaining. Scale bar, 5 μm. ( f ) Total airway epithelial cell numbers per millimeter basal lamina at 0 days (baseline) and at 12 days post LPS instillation. Bars=group means±s.e.m. ( n =>3 mice/group); * P <0.05. Full size image To test whether this effect is observed in the C57Bl/6 background that is considered most resistant to developing mucous cell metaplasia, we backcrossed the p53 TTAA , p53 ΔP and p53 AXXA mice that were generated on the 129J background into C57Bl/6 background over at least 10 generations. Results showed that in 129J and C57Bl/6 mice the mutations in the p53 PRD also increased the number of mucous cells per mm basal lamina ( Fig. 6c ), suggesting that this genotype drives mucous differentiation irrespective of the more resistant genetic pool present in C57Bl/6 mice. In addition, immunostaining with Muc5ac antibodies showed that tissue sections from p53 AXXA , p53 TTAA and p53 ΔP mice compared with p53 wt exhibited significantly more positivity for Muc5ac ( Fig. 6d ). Further, Bcl-2- and Muc5ac-positive cells in p53 AXXA compared with p53 WT mice are higher at 12 days after LPS instillation ( Fig. 6e ). While the total cell number per mm basal lamina is similar in p53 WT and p53 AXXA 12 days after LPS challenge, the hyperplastic changes remain in p53 AXXA but not in p53 WT mice ( Fig. 6f ). These findings suggest and show that the p53 PRD is central in regulating mucous metaplastic changes at baseline and during the resolution of hyperplastic changes. The present study defines the PRD of p53 as a crucial region that affects regulation of SPDEF and Bcl-2 to drive the mucous hypersecretory phenotype in humans and in rodents. Within the PRD of p53, substitution of Pro in the PVAP motif to Arg or Ala or modification of Thr to Ala was sufficient to increase both SPDEF promoter activity and bcl-2 mRNA half-life and drive the mucous regulatory network at baseline and to sustain the mucous cells following a hyperplastic response. It is generally believed that under physiological conditions, apoptosis induction by p53 mainly depends on the transcription of a distinct set of cell death regulatory genes. p53 is a major transcription factor that affects numerous promoter regions [43] . The DNA-binding region of p53 is the main region to affect transcription of genes known to directly execute apoptosis including the TNF-R family members, such as CD95/Fas/Apo-1, DR4 and DR5/TRAIL-R1, and the Bcl-2 family members, such as Bax, Puma, Noxa and Bid [44] . However, the present studies show that the PRD of p53 also enhances cell death by reducing bcl-2 mRNA half-life through interactions with the 5′UTR region and suppressing expression of this central inhibitor of apoptosis. Despite the previous reports that interaction of p53 with the P2 promoter region suppresses P2 promoter activity in primary airway and lung cancer cell lines [7] , [9] , we first suspected that p53 does not suppress bcl-2 promoter activity when we noticed that within the context of the full-length P1-M-P2 promoter. First, the extent of this suppression was not sufficient to explain the drastic reduction in Bcl-2 protein when p53 is activated and the P2 promoter region was able to suppress the P1-M promoter activity independently of p53. These observations led us to hypothesize that p53 affects bcl-2 mRNA stability instead. We found that P2 sequences are part of the 5′UTR of bcl-2 transcripts, which is consistent with previous studies reporting that P2 initiates a small percentage of transcripts in cells such as B cells [45] . Because of their extremely labile nature, as evidenced by the smears observed in Northern blot analyses [11] , [12] , [45] , previous attempts to characterize all the bcl-2 mRNA transcripts by techniques such as the S1 nuclease assay may not have been sufficiently sensitive. Although we also found the previously identified T2, a transcriptional start site located within the GC-rich region at −1,313 (ref. 11 ), the other transcriptional start sites, T1, T3 and T4 have previously not been reported. All these transcripts contain a region of P2 that affects mRNA stability. The p53 interaction with the 5′UTR of bcl-2 mRNA was demonstrated by the following studies: (1) all four bcl-2 transcripts were precipitated from cell extracts with p53 antibodies; (2) p53 was detected in pull-down assays using in vitro synthesized bcl-2 mRNA; (3) p53 Pro more drastically than p53 Arg destabilized endogenous bcl-2 mRNA and luciferase mRNA that was expressed from the P1-M-P2 luciferase constructs and (4) deletion or mutations of a 16-nucleotide region of P2 prolonged the luciferase mRNA half-life, demonstrating that p53 reduces bcl-2 mRNA half-life by interacting with this 16-nucleotide region within the 5′UTR. Previous studies have found that the AU-rich elements (AREs) in the 3′UTR of bcl-2 mRNA can bind AUF1 and TINO that cause a two-fold destabilization of the mRNA [46] , [47] or Bcl-2 protein itself that is required for ARE-dependent degradation of its own mRNA [46] . Nucleolin, another protein that interacts with the AREs, stabilizes the bcl-2 mRNA [48] . The p53-mediated decay required only the 5′UTR but is independent of the 3′UTR of bcl-2 mRNA. The p53 Pro variant may be more efficient than the p53 Arg variant in forming a macromolecular complex that helps recruit RNA enzymes to target bcl-2 mRNA. We searched both the genome and transcriptome for exact matches to the 16 nucleotides that were important for the interaction and enhanced decay of bcl-2 mRNA. Two other exact matches were found in the genome, and both reside ~37.5 kb away from the FRG2 and FRG2B genes on chromosomes 4 and 10, respectively, but neither of these positions are transcribed regions. No exact matches, other than in the bcl-2 5′ UTR, were found in a search of all RefSeq and GenBank mRNAs. Mutation of 4 nucleotides on either end of the 16 nucleotides did not fully stabilize the bcl-2 mRNA, although these changes abolished interaction of p53 from cell extracts. These findings suggest that secondary structures of the bcl-2 mRNA rather than a specific nucleotide sequence may be important for interaction with p53. The participation of factors that may bind to P2 sequences and form a scaffold for p53 interaction are yet to be identified. One previous study has reported that p53 binds to the 5′ UTR of cdk4 to inhibit TGF-beta-regulated translational of cdk4 [49] . The similar half-life of bcl-2 mRNA in HAECs and p53-deficient H1299 cells suggests that the function of p53 to enhance decay is tightly regulated. In addition, the need to activate p53 by UV irradiation to reduce bcl-2 mRNA half-life in HAECs implies that either only activated p53 can interact with bcl-2 mRNA or that other factors may facilitate this interaction. A wide range of cellular stresses, such as DNA damage, telomere erosion, aberrant oncogene activation or hypoxia, causes p53 accumulation and activation, indicating that protein abundance may dictate function [10] . The observation that bcl-2 mRNA half-life in A549 cells was reduced without inducing a cellular stress response supports that p53 is either constitutively activated in these cells in regard to destabilizing bcl-2 mRNA or that the factor(s) required for p53 interaction with bcl-2 mRNA are present. However, as p53 levels are low in A549 cells, we speculate that post-translational modifications such as phosphorylation of various serine and threonine residues, acetylation and methylation of specific p53 domains [50] and/or cooperation with other transcription factors [51] may be responsible for the interaction to enhance the decay of bcl-2 mRNA. Modifying p53 expression in both SAOS-2 and HCT116 cells or simply substituting the proline or threonine residues within the PRD of p53 affected bcl-2 mRNA levels and mRNA half-life in human and murine cells. The fact that it is not only the substitution of the conserved PXXP motif but also the substitution of threonines with alanines affecting the decay of bcl-2 mRNA across cell types and species suggests that it is the conformational change that is introduced by any modification within the PRD to be the primary cause for the ability of p53 to interact with higher affinity to SPDEF promoter or bcl-2 mRNA. The PRD lies within the N-terminal region of p53 (aa 61–94) and is characterized by two transactivation domains that are required for transcriptional activation of target genes [50] . Previous studies have focused on the contribution of the PRD to the regulation of p53 stability, transactivation ability and induction of transcription-independent apoptosis [32] , [33] , [52] . p53 Pro activates expression of certain genes by binding more strongly to TAFII70 and TAFII32, major components of the basic transcriptional machinery, than does p53 Arg (ref. 33 ). That p53 Arg compared with p53 Pro interacts stronger with both the P2 sequences of the bcl-2 mRNA and the SPDEF promoter is consistent with those observations. Consistent with our findings, a previous study had reported that Bcl-2 immunopositivity tended to be more in tumours with the p53 Arg variant [53] . However, the present studies are the first to link the PRD of p53 to regulating mRNA stability. At baseline, p53 AXXA mice show increased metaplastic mucous cells compared with p53 WT mice, while the total airway epithelial cell numbers are similar, likely due to increased SPDEF levels. However, after LPS instillation that caused a hyperplastic response equally in p53 +/+ and p53 −/− mice, the resolution of hyperplasia was intact in p53 +/+ mice but was disrupted in p53 −/− and p53 AXXA mice. The induction of mucous expression in mice instilled with LPS is independent of SPDEF, as during such inflammatory responses IL-1β [54] and neutrophil elastase [55] cause increased expression of Muc5ac and Bcl-2 (ref. 15) . However, sustained hyperplasia in p53 −/− and p53 AXXA mice is likely due to increased Bcl-2 expression in these mice. When transcription is blocked with 5,6-dichloro-1-beta- D -ribobenzimidazole (DRB), p53 Pro more efficiently causes cell death than p53 Arg due to drastically reduced Bcl-2 levels caused by the high bcl-2 mRNA decay rate by p53 Pro . The finding that cyclohexamide- or thapsigargin-induced cell death equally well in both H1299p53 ts Arg and H1299p53 ts Pro cells when co-treated with DRB may suggest that Bcl-2 does not affect protein shutdown- or ER-induced cell death but DNA damage-induced cell death caused by doxorubicin, UV irradiation, hyperoxia or hypoxia. Cell-type differences in apoptotic pathways induced by p53 Arg and p53 Pro may explain the findings that the p53 Pro was found to be less apoptotic [56] . Findings from our studies suggest that using a combination of DNA polymerase II inhibitors to enhance bcl-2 mRNA decay along with radiation and chemotherapy may better target cancers of individuals harbouring the p53 Arg genotype rather than using DNA damaging agents only. While the association of the p53 polymorphisms with cancer incidence is inconclusive, several studies have suggested that individuals homozygote for p53 Arg have a better response and survival rate following chemo- and radiation therapy for head and neck, breast and lung cancers (reviewed in ref. 57 ). The effect of this SNP on the mucous differentiation pathway is highly conserved, suggesting that these mice with modifications in the PRD of p53 closely reflect the susceptibility in humans and should be most appropriate for screening potential drugs to treat CMH. Many drugs that are screened in mice fail in human trials because of vast differences in pathways. Testing potential drugs in mice that replicate the disease in humans, such as the p53 AXXA mice, not only would help in improve design but also increase the likelihood of success in human clinical trials. Similar strategies that use genetically engineered mouse models have shown success in predicting the outcome of clinical trials [58] , [59] . Study population The LSC (Lovelace Smokers’ Cohort) is a well-characterized cohort of current and former smokers in New Mexico. Recruitment, inclusion and exclusion criteria have been described previously [60] , [61] . In brief, study subjects were drawn from a cohort study Albuquerque, NM and its surrounding communities. Most participants were recruited through newspaper or television advertisements and were paid a small stipend for their participation. Subjects were included in the study if they were ages 40 to 75 years, former or current smokers with a minimum smoking history of 20 pack-years on initial screening and able to understand English. Information related to demographics, respiratory diseases and smoking was obtained by self-report from all study participants via a questionnaire. Spirometry was obtained on all subjects by certified and registered respiratory therapists strictly adhering to the 1994 American Thoracic Society (ATS) guidelines. The LSC disproportionately enrolled women ever-smokers as the disease prevalence from 1998 onwards is significantly higher among women than men [62] and as women are under-represented in most COPD studies in the United States [63] . This study is approved by the Western Institutional Review Board (Olympia, WA; #20031684) and all subjects sign informed consent for their participation. Animals Pathogen-free wild-type 129J and C57BL/6J mice and p53 −/+ breeders were purchased from The Jackson Laboratory (Ben Harbor, ME). p53 wt , p53 AXXA , p53 TTAA and p53 ΔP mice on 129J background were provided by Dr Geoffrey M. Wahl (Salk Institute for Biological Studies, LaJolla, California). Mice were housed in isolated cages under specific pathogen-free conditions and bred at LRRI for the described studies. The p53 ΔP mice were genotyped by standard PCR that show different products from wild-type mice, and the AXXA and TTAA mice were genotyped using restriction digestion of PCR amplified products to distinguish the knock-in from wild-type mice (primer sequences can be found in Supplementary Table 3 ). These mice were also backcrossed for at least 10 generation into the C57BL6 background. Right cranial lung lobes were removed from mice and tissue homogenized using TissueLyser II (Retsch, Newtown, PA) and RNA isolated and qRT-PCR performed as described previously [29] . Mice were randomized by weight for each study. p53 +/+ and p53 −/− mice were intransally instilled with 60 μg LPS as described [29] . Left lungs were inflated and fixed at 25 mm pressure with zinc formalin for preparing tissue sections, which were stained with Alcian blue (AB), haematoxylin (H) and eosin (E) or were immunostained. Images were captured using NanoZoomer Digital Pathology slide scanner (Hamamatsu, Bridgewater, NJ) and epithelial and mucous cells quantified using Visiopharm Integration System (VIS) software (Horsholm, Denmark). For all mice, epithelial cells in the axial airway of the left lung at generation 4 or 5 are quantified. A minimum of three adult mice were used for isolation of MAECs that were cultured for differentiation on Transwell inserts according to described methods [64] . All experiments were approved by the Institutional Animal Care and Use Committee of Lovelace Respiratory Research Institute (LRRI) and were conducted at LRRI, a facility approved by the Association for the Assessment and Accreditation for Laboratory Animal Care International. Cells Primary HAECs from individuals homozygous for the p53 Arg and p53 Pro variants were obtained from lungs under the protocol and consent form approved by the University of North Carolina School of Medicine Committee on the Protection of the Rights of Human Subjects. HAECs from each individual and those purchased from Clontech (Walkersville, HD), and AALEB cells (Immortalized and transformed HAECs) [65] were maintained in BGEM media (Cambrex Biosciences, Walkersville, HD) with various supplements as described [66] . After seeding primary HAECs on Transwell membranes and differentiating them on ALI, membrane quarters were used for qRT-PCR and membrane halves embedded in paraffin. Sections were stained with AB/H&E and imaged with Nikon (Irvine, CA) E600 light microscope and × 40 images captured with Nikon DXM1200F camera using ACT-1 software. Epithelial and mucous cells quantified using Visiopharm Integration System (VIS) software. SAOS-2 (human osteosarcoma cell line, ATCC HTB-85), Calu-3 (human lung Adenocarcinoma cell line, ATCC HTB-55), H23 (NCI-H23, lung Adenocarcinoma, ATCC CRL-5800), HBEC-2 (human immortalized airway epithelial cells) and A549 (immortalized and transformed human alveolar cells, ATCC CCL-185) cells were maintained in Dulbecco’s modified Eagle’s media (DMEM) supplemented with 10% FBS. Expression vectors for p53 Arg or p53 Pro variants at codon 72 have been shown to induce cell death differentially in SAOS-2 cells [56] . The H1299 cell line (NCI-H1299, ATCC CRL-5803), a p53-deficient cell line that is derived from a non-small cell lung cancer, was used to generate stable cell lines by transfecting with pCMV-neo-bam tsp53 Arg72 or pCMV-neo-bam tsp53 Pro72 plasmids (gift from Dr Murphy, University of Pennsylvania, PA) that express temperature-sensitive p53 variants. These variants are essentially inactive at 37 °C but are activated when cells are shifted to 32 °C. Clones expressing similar p53 protein levels were selected for further experiments (see Supplementary Fig. 5 ). H1299 cells and those harbouring temperature-sensitive p53 variants for Arg and Pro at codon 72 were maintained in RPMI-40 (Gibco) with 10% FBS, and 2 mM glutamine, and 400 μg ml 1 G418 (Sigma Chemicals). Mouse embryonic fibroblasts (MEFs) from p53 wt , p53 ▵ P , p53 TTAA and p53 AXXA mice were derived from day 14.5 to 16 embryos, and were cultured in DMEM supplemented with 10% FBS and were used for experiments at passages 3–8. MEFs were infected (10 MOI) with adenoviruses expressing p53 Arg or p53 Pro . Twenty-four hours later, cells were washed and treated with 1 μM doxorubicin for 24 h. Cells were counted and harvested for western blot analyses. SAOS-2 cells stably transfected with either p53-expressing plasmid (SAOSp53) or vector only (SAOS-2Ctr) were a gift from Dr Michael Resnick (National Institute of Health Environmental Sciences; Dallas, TX) and were maintained in DMEM supplemented with 10% FBS and 0.5 mg ml –1 G418. Cell death assay Following treatment with 50 ng ml −1 DRB and 1 μM doxorubicin, 10 μM cyclohexamide or 1 μM thapsigargin, viable cell numbers were quantified using trypan blue exclusion method. Cells were also irradiated with 10 mJ UV light, were treated with hypoxia (5% O 2 /95% nitrogen) or hyperoxia (95% O 2 /5% nitrogen) for 30 m at room temperature and were cultured at 37 °C in an incubator with 5% CO 2 /95% air. Cells were harvested 24 h after treatment by trypsinization and cell numbers were quantified using trypan blue exclusion method. For AnnexinV-PI staining, ~10 5 cells were also stained in 1X binding buffer (0.01 M HEPES, pH 7.4; 0.14 M NaCl; 0.25 mM CaCl 2 ) using 5 μl propidium iodide (Sigma) and 10 μl of Annexin V-FITC (BD PharMingen). The reaction was incubated in the dark for 15 min at room temperature and the percentage of FITC- and PI-positive cells were collected on FACS Canto (BD Biosciences; San Jose, CA) flow cytometer and analyzed using FlowJo software (ver 7.6.3; TreeStar, San Carlos, CA). Generating deletion constructs and site-directed mutagenesis The generation of the P1-M-P2 luciferase construct has been described previously [7] , and the P1-M-P2 constructs in which P2 was serially deleted (P1-M-P2Δ1-10) were generated by amplifying the P2 region with primers listed in Supplementary Table 1 that introduced the upstream Bgl-II and a downstream Hind-III site. The amplified products were then used to replace the full-length P2 sequence that was removed by restriction digestion using Bgl-II and Hind III. For in vitro mRNA synthesis, the P1-P2Δ10 luciferase construct was cloned in to PCRIITOPO vector (Invitrogen) that has the dual promoter system for REMSA. The 50-nucleotide-long forward and their reverse oligonucleotides sets were designed having the Xba-I in the upstream sequence and Hind-III restriction site on the downstream sequence. The 16-nucleotide sequences with putative p53-interaction sites were mutated by changing the purines to pyrimidines as shown by the underlined sequences in Supplementary Table 2 . The oligonucleotides were annealed, double-stranded DNA generated, and following digestion with Xba-I and Hind-III restriction fragments were cloned into a pCR-II dual promoter vector. These plasmids were then used for in vitro transcription (IVT) and pull-down using a 1:500 diluted p53 antibody (sc-98, Santa Cruz Biotechnology, CA). Two deletion mutants were generated in the dual promoter vector, pCR-2.1, harbouring the P2 region using Quickchange site-directed mutagenesis kit (Stratagene) according to the manufacturer’s protocol. The resulting mutant constructs, pCR-2.1 P2(−482/−468) and PCR-2.1 P2(−443/−429), in which 16 and 14 nucleotides, respectively, had been deleted were used for IVT synthesis and pull-downs using the p53 antibody (sc-98, Santa Cruz). The P1MP2Δ(−443/−429) luciferase construct in which 16 nucleotides were deleted from P1MP2 luciferase plasmid and PIMP2Δ(−443/−439 and −433/−429) were generated at Mutagenex (Somerset, NJ). These deleted plasmids were used for transient transfection in HCT116 p53 positive cells to determine the effect of this deletion on luciferase mRNA half-life. Both SPDEF promoter deletion mutants (Mut11 and Mut21) were also generated at Mutagenex. RNA extraction and RT-PCR Total RNA was extracted from Calu-3, A549, AALEB, SAOS-2, H1299, HBEC-2, NHBEC and transfected H1299 cells using TRI reagent (TR-118; Molecular Research Centre, Inc.) as described by the manufacturer. For cDNA synthesis, 1 μg of total RNA or RNA treated with RNAse free DNase (Invitrogen) was reverse transcribed with Random Hexamers (Promega). Primers with the following sequences: M Forward: 5′- GCAGGACCAFFAGGAGGAGA -3′, M Reverse 5′ GGTGG GGGAGG TTTTATTT -3′, and P2 Forward: 5′- CGATC TGGAAATCCTCCTAATT -3′ and P2 Reverse: 5′- TTGGCATGAGATGCAGGAAA -3′ were designed to amplify the M and P2 regions of the bcl-2 promoter. After denaturing at 95 °C for 5 min, reactions were amplified for 35 cycles using annealing temperatures of 55 °C for M primers and 60 °C for P2 primers. 5′Rapid Amplification of cDNA Ends (RACE) To identify the 5′UTR, we used the rapid amplification of cDNA ends (RACE) kit (Invitrogen; San Diego, CA) on RNA isolated from HAECs according to the manufacturer’s instructions. In brief, total RNA (5 μg) was dephosphorylated with 10 U μl −1 calf intestinal phosphatase (CIP) and treated with 0.5 U μl −1 tobacco acid phosphatase (TAP) to remove the 5′ CAP structure. The 5′gene racer oligo was ligated to the RNA using T4 RNA ligase and the first strand cDNA was synthesized using random hexamers and superscript III RT. Transcripts were identified by PCR using the gene racer primer R1 and primers specific to the M region (M1: 5′ GTGGGGGAGGTTTTATTT -3′) or bcl-2 ORF (ORF1: 5′ CGCTGGGAGAACAGGGTACGATAA -3′). Amplification using nested racer primer R2 and gene-specific primers specific to the M region (M2: 5′- ATGACTGCTACGAAGTTCTCCC -3′) and the bcl-2 open-reading frame (ORF2: 5′- TGGCGCACGCTGGGAGAACA -3) were used to ensure specificity of products, followed by cloning into TOP10 vector (Invitrogen, CA) for sequencing. mRNA half-life studies Following treatment with the transcription inhibitor 5,6-dichloro-1-beta- D -ribobenzimidazole (DRB) (Sigma-Aldrich), total RNA was extracted using TRIzol reagent. RNA levels were normalized using 18S rRNA and GAPDH amplified from the same RNA samples using Pre-Developed 18S rRNA (VIC-MGM) and hGAPDH (ABI Assay-on-Demand FAM-MGM probe). Relative mRNA abundance was calculated using the ▵ ▵ Ct method and mRNA half-life was calculated as described [42] . The primers and probe for detecting luciferase mRNA expression by qRT-PCR were LUCForward 5′- ACCTCCGTACTATCCTTTGGAAGAA -3′ LUCReverse- 5′- GGAACTGCGGCATATCGTGATA -3′ and the probe sequence with the dye LUC-FAM-5′- ACTGCGGGAGAACAA -3′. Western blot analysis Cell extracts were prepared using RIPA buffer (20 mM Tris, pH 7.4, 137 mM NaCl, 1% NP-40, 0.25% Deoxycholate, 0.1% SDS, 1 mM EDTA and 1% protease inhibitor cocktail). Protein concentration was determined by BCA kit (Pierce; Rockford, IL) and 100 μg protein was analysed by western blotting as described previously [67] . Anti-p53 (sc-98, Santa Cruz) was used at 1:1,000 (2 μg ml −1 ) dilution and anti-Bcl-2 (sc-492, Santa Cruz) and anti-β-actin (Sigma) were used at 1:1,000 dilutions. SPDEF antibodies (gift from Dr Jeffery Whitsett, Children’s Hospital, University of Cincinnati, OH) were used at 1:5,000 dilution. Proteins were detected using ECL and visualized by chemiluminescence (Perkin Elmer, Waltham, MA) using the FujiFilm Image Reader LAS-4000 (Valhalla, NY). The uncropped scans of the most important western blots are included as a Supplementary Figure in the Supplementary Information . Co-immunoprecipitation assays Immunoprecipitation of protein-RNA complexes was performed as described previously [68] . H1299p53 ts cells (8 × 10 7 ) were incubated at 32 °C, harvested, and proteins cross-linked using formaldehyde (Sigma) at a final concentration of 0.5% (v/v) and incubated at room temperature for 10 min. Cross-linking was quenched with glycine (pH 7.0, 0.25 M final concentration), and cells were lysed with three rounds of sonication in 1 ml of RIPA buffer containing protease inhibitors. An aliquot of the cell lysate (500 μl each) was mixed with 20 μl of protein-A Sepharose beads for 1 h at 4 °C followed by centrifugation at 400 g for 5 min. The pre-cleared supernatant was diluted with RIPA buffer (250 μl) containing RNAsin and protease inhibitors, mixed with polyclonal anti-p53 (0.2 μg μl −1 ) (sc-98, Santa-Cruz) or IgG (0.2 μg ml −1 ) and incubated overnight at 4 °C with slow mixing. Protein-A Sepharose beads (100 μl) were added to the samples followed by incubation at 4 °C for 3 h. The Sepharose beads were washed five times with RIPA buffer, beads were centrifuged for 5 min at 200 g and mRNA-protein complexes eluted with 120 μl hot SDS and boiled for 5 min. Beads were incubated at 70 °C for 45 min to reverse cross-linking and then centrifuged for 5 min at 13,000 g and eluted. From both p53 and IgG 1 , 20 μl samples were removed for western blot analysis. RNA was extracted from the remaining samples using TRIzol (Invitrogen) according to the manufacturer’s protocol, treated with DNAse I and used as a template for qRT-PCR using probe and primer set for human Bcl-2 (ABI Assay-on-Demand FAM-MGM probe) and to synthesize cDNA using random hexamer primers (OmniScript Invitrogen). PCR was performed using 5 μl of the cDNA samples using primer sets for the four transcripts: T1 Forward: 5′- CCTGC CGCGG CGCCT TTAAC -3′ Reverse: 5′- ATGAC TGCTA CGAAG TTCTCCC -3′, T2 Forward: 5′- GCAGG ACCAG GAGGA GGAGA -3′ Reverse: 5′- GGTGG GGAGG TTTTATTT -3′. T3 Forward: 5′- CGATC TGGAA ATCCT CCTAATT -3′ Reverse: 5′- TTGGC ATGAG ATGCA GGAAA -3′ and T4 Forward: 5′- TGGGG TGGGA GCTGG GGCGA -3′ Reverse: 5′- CCCCC GTTGC TTTTCCT -3′ regions of the Bcl-2 5′UTR region. Chromatin-immunoprecipitation assay H1299 cells harbouring temperature-sensitive p53 Arg or p53 Pro variants, and MEFs from p53 WT and p53 AXXA cells were used for ChIP assays as described previously [42] . In brief, cells were fixed with 1% formaldehyde, and the reaction was quenched using 1.25 M glycine and scraped into cold PBS containing protease inhibitors. ChIP was performed using the Magna ChIP G kit (MAGNA0002; EMD Millipore) as described by the manufacturer. Sonicated nuclear fractions were incubated with the p53 antibody using mouse monoclonal (sc-98, clone Pab1801; Santa Cruz Biotechnology) and rabbit polyclonal (sc-6324, clone FL393; Santa Cruz Biotechnology) for human and murine p53, respectively. DNA identification was confirmed with PCR using the following primers specific for the human and murine SPDEF promoter regions: 5′- CTGATCCATCTTAGAACCCCAGCCC -3′ (forward), and 5′- GGATCCATGCCCTGACAGCTAGG -3′ (reverse); and 5′- GGAGAGAGAACTCAGCAGTTAAG -3′ (forward) and 5′- GTGTCACCACACCTGACTATC -3′ (reverse), respectively. The 4 and 6 kb upstream for human and murine SPDEF regions, respectively used the following specific primers: 5′- CTGTGAGTGAGACAGGCAATGACCC -3′ (forward) and 5′- TTGGGACCAGAGAGGCTAGGGAC -3′ (reverse); and 5′- GTTTGACTCTCTCCTGGCTTTC -3′ (forward) and 5′- CATCTACTAC ACGCCAAGTT CC (reverse), respectively. In-vitro RNA transcription and RNA pull-downs Biotinylated RNA transcripts were synthesized using the in vitro transcription kit from Enzo Life sciences (Farmingdale, NY) as described by the manufacturer. In brief, reactions were performed using T7 (sense) and SP6 (antisense) promoters to synthesize P2 RNA from pCR-2.1 P2. In vitro transcription (IVT) reactions contained 1 μg of linearized plasmid template treated with Proteinase K (100 μg ml −1 ) and 0.5% SDS and reaction incubated for 30 min at 50 °C. After phenol/chloroform extraction, DNA was precipitated overnight by adding ethanol. DNA was resuspended in RNAase/DNAase-free water (Hyclone, Thermo Scientific, Logan, UT) and incubated with transcription reaction for 1 h at 37 °C, before treatment with RNAse-free DNAse-1 (Turbo, Enzo Life Science, Farmingdale, NY). Biotin-labelled probes were purified by precipitating with 4 M LiCl and 100% ethanol. The RNA pellet was dissolved in 2 × TEN (20 mM Tris-HCL pH 8.0, 2 mM EDTA pH 8.0 and 500 mM NaCl) and quantified. Cytosolic S-100 extract was prepared using H1299p53ts cells incubated at 32 °C. Cells were washed twice in cold PBS and then suspended in 500 μl of buffer D (10 mM Hepes (pH 8.0), 3 mM MgCl 2 , 40 mM KCl, 0.1% protease inhibitor cocktail (Sigma), 0.2% NP-40 (Nonidet P40), 10% glycerol, and 1 mM DTT (dithiothreitol) and incubated on ice for 10 min. The cells were lysed with 50 bursts using a Branson sonifier 25 sonicator (Thomas Scientific). The lysate was centrifuged at 10,000 g for 2 min to pellet nuclei, followed by centrifugation at 20,000 g for 1 h at 4 °C to produce the cytosolic S-100 extract. IVT RNA was incubated with 300 μg of S-100 extract in 2X TENT buffer (20 mM Tris-HCL pH 8.0, 2 mM EDTA pH 8.0, 500 mM NaCl and 0.5% v/v Triton X-100) for 30 min at room temperature with gentle mixing. Pull-downs were performed in the presence of 1% Triton X-100 using Dynabeads M-280 cross-linked to steptavidin beads (Invitrogen). Each pull-down reaction was incubated with 300 μg of S-100 extract and Dynabeads for 30 min at room temperature with gentle mixing. Dynabeads were settled with magnetic beads and centrifuged for 5 min at 1,000 g . The RNA–protein–bead complexes were washed three times, eluted with 30 μl hot SDS and pull-down products analysed for p53 by western blotting. The ChIP assay was performed as we have described [42] . Gene silencing in differentiated HAECs Differentiated HACEs were transduced with retroviral expression vectors for Bcl-2 shRNA, SPDEF shRNA and control shRNA (Origene Technologies, Inc., Rockville, MD) as per the manufacturer’s instructions. Transwell membranes were harvested and expression of certain genes analysed by qRT-PCR and western blot analyses. Statistical analysis Grouped results from at least three or four different sets of experiments were expressed as mean with s.e.m., and differences between groups were assessed for significance by Student’s t -test when data were available in only two groups. When data were available in more than two groups, analysis of variance (ANOVA) was used to perform pair-wise comparison. When significant main effects were detected ( P <0.05), Fisher least significant difference test was used to determine the differences between groups. A P -value of 0.05 was considered to indicate statistical significance. The difference in the mean ΔCT values from qRT-PCR amplifications between the two homozygote genotypes of HAECs was assessed with a two-sample t -test. Both, the difference and the difference plus one s.e. were summarized by expressing as fold change. How to cite this article: Chand, H. S. et al . A genetic variant of p53 restricts the mucous secretory phenotype by regulating SPDEF and Bcl-2 expression. Nat. Commun. 5:5567 doi: 10.1038/ncomms6567 (2014).